Pseudogap in a thin film of a conventional superconductor A superconducting state is characterized by the gap in the electronic density of states, which vanishes at the superconducting transition temperature T c . It was discovered that in high-temperature superconductors, a noticeable depression in the density of states, the pseudogap, still remains even at temperatures above T c . Here, we show that a pseudogap exists in a conventional superconductor, ultrathin titanium nitride films, over a wide range of temperatures above T c . Our study reveals that this pseudogap state is induced by superconducting fluctuations and favoured by two-dimensionality and by the proximity to the transition to the insulating state. A general character of the observed phenomenon provides a powerful tool to discriminate between fluctuations as the origin of the pseudogap state and other contributions in the layered high-temperature superconductor compounds. Superconductivity, that is, the ability of certain materials to carry loss-free current, appears because of the interaction of conducting electrons with the vibrational motion of atoms [1] . The mediating action of atomic vibrations induces attraction between the electrons with the opposite spins and momenta, and causes them to combine into bound pairs called Cooper pairs. Being bosons, Cooper pairs condense at the lowest possible quantum state. To break a Cooper pair and remove the two resulting unbound electrons from the condensate, one has to spend the energy 2Δ, the quantity Δ being called as the superconducting gap. This means that the gap 2Δ appears in a single electron density of states (DOS). This gap in the DOS is characteristic of a superconducting state and vanishes above the superconducting transition temperature T c . However, high-temperature copper oxide-based superconductors exhibit a considerable suppression in the DOS over a wide range of temperatures above T c , as evidenced by nuclear magnetic resonance, infrared conductivity, neutron scattering, transport properties, specific heat, thermoelectric power, spin susceptibility, Raman spectroscopy, tunnelling conductance data and angle-resolved photoemission [2] , [3] , [4] , [5] . This 'pseudogap' has become the focus of the condensed matter community, as it is viewed as a key to understanding the nature of high-temperature superconductivity [6] . A possible way of understanding the pseudogap phenomenon follows from the pioneering work [7] by Anderson who proposed that high- T c superconductivity stems from the copper oxides being Mott insulators well above T c (ref. 8 ). The same enhanced electron–electron interaction that turns the material insulating favours electron pairing. Accordingly, from this viewpoint, the pseudogap reflects the massive presence of paired electrons above T c and transforms into a superconducting gap below T c . Within the standard Bardeen–Cooper–Schrieffer theory, the stable Cooper pairs are energetically advantageous at temperatures below T c (ref. 1 ). Short-living fluctuation-induced pairs can appear even at T > T c (refs [9] , [10] 9,10). However, in clean bulk conventional superconductors, the range of temperatures in which superconducting fluctuations (SFs) are important is extremely narrow, that is, about δT ~10 −12 to 10 −14 T c . Effects of fluctuations are favoured by disorder and by lowering the dimensionality of the system; in the context of superconducting films, the latter condition implies that the thickness of the film is less than the superconducting coherence length ξ . The relevance of fluctuations is quantified by the Ginzburg–Levanyuk parameter, which in two-dimensional disordered systems is Gi = δT/T c ≈( e 2 /23ħ) R , the sheet resistance R characterizing the degree of disorder. Accordingly, fluctuations gain importance in high-temperature copper oxide compounds that are made up of parallel two-dimensional conducting sheets containing copper and oxygen atoms and sandwiching in between atoms of other kinds. Note at the same time that reduced dimensionality promotes not only superconductivity but also a competing effect, the localization. Thus, increasing the sheet resistance by doping can drive bulk cuprates across the superconductor–insulator transition (SIT) into an insulating state [11] , [12] , [13] , [14] . At the same time, underdoped superconductors exhibit an appreciable growth of the temperature range of the existence of the pseudogap on approaching the SIT, that is, on increase of the sheet resistance [2] . In general, analysing a wealth of experimental data collected during the past decade, we observe a remarkable similarity between the behaviours of the underdoped copper oxides and thin disordered films of conventional superconductors near the SIT, although important differences remain, such as the anti-ferromagnetic order of the cuprates, deep in the insulating side of the SIT. This heralds that an understanding of pseudogap is to be gained through identifying parallels across different classes of superconductors, and makes quasi-two-dimensional films of conventional superconductors the exemplary model systems for seeking the pseudogap physics because of the presence of paired electrons above T c . If the pseudogap is induced by superconducting pairing above T c , one would expect that two-dimensional superconducting films should exhibit it as well. In this article, we show that a pseudogap indeed exists in conventional disordered superconducting films far above T c . Furthermore, the quantitative analysis of the thermal evolution of the DOS demonstrates the SF-origin of this pseudogap. Disordered thin films as a testing ground for correlated physics Our study of the ultrathin (5 nm thick) titanium nitride (TiN) films in search of the pseudogap-like behaviour is motivated by all the issues mentioned in the previous section. The coherence length in these films, ξ =10 nm (ref. 15 ), is much larger than the film thickness, thus ensuring that they are two-dimensional superconductors. Our recent research revealed that the 5-nm-thick TiN films exhibit a SIT that can be traversed either by changing the strength of disorder [16] , [17] , the tunable measure of which is the room temperature resistance, or by the external magnetic field [15] , [18] . The choice of TiN films is supported by recent findings of a mid-infrared feature in their optical conductivity [19] , which is reminiscent of a pseudogap-like excitation in cuprates [4] . The observed suppression of T c with increasing R ( Fig. 1a ) signals the enhancement of Coulomb effects [20] , [21] . In clean superconductors, the charge carriers move freely and react instantaneously to fluctuations of the electric fields, eliminating Coulomb interactions on the distances exceeding the atomic spatial scales. This ideal screening permits the phonon-mediated Cooper pairing and makes the very phenomenon of superconductivity possible. Disorder impedes the motion of electrons, which then lag behind the alternations in the distribution of the electric field caused by changes in their mutual spatial positions. This breaks down the dynamic screening of Coulomb interactions, and the electron–electron Coulomb repulsion starts to come into play. Thus, the impaired screening ignites the competition between Coulomb forces and superconducting pairing, effectively decreasing the strength of the Cooper electron–electron attraction. 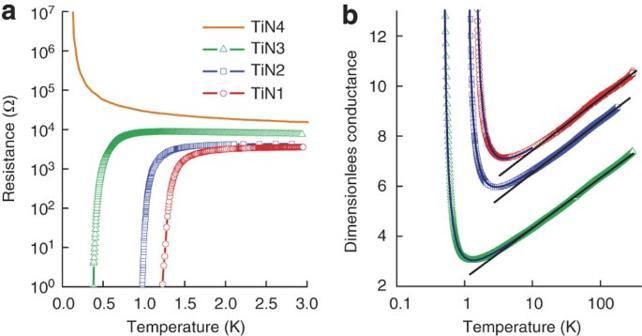Figure 1: Transition to a superconducting state of the TiN films. (a) Sheet resistance versus temperature plots of TiN films at low temperatures. As the resistance at room temperature grows, the critical superconducting temperatureTcdecreases (the plots for samples TiN1 to TiN3 were published in ref.22in a different form) and the sample TiN4 becomes insulating at low temperatures. (b) The same data as ina, but extended to room temperatures and re-plotted as the dimensionless conductanceg=(h/e2R). The semi-logarithmic representation reveals logarithmic decrease of the conductance with temperature owing to weak localization and Coulomb interaction effects. The black straight lines highlight this behaviour. Transition temperatures equal to 1.3, 1.0 and 0.45 K for TiN1, TiN2 and TiN3, respectively, are obtained by fitting the conductance curves with all the quantum corrections to the conductivity. The fitting procedure is described in the Methods. The fits are shown as solid curves. Figure 1: Transition to a superconducting state of the TiN films. ( a ) Sheet resistance versus temperature plots of TiN films at low temperatures. As the resistance at room temperature grows, the critical superconducting temperature T c decreases (the plots for samples TiN1 to TiN3 were published in ref. 22 in a different form) and the sample TiN4 becomes insulating at low temperatures. ( b ) The same data as in a , but extended to room temperatures and re-plotted as the dimensionless conductance g =( h / e 2 R ). The semi-logarithmic representation reveals logarithmic decrease of the conductance with temperature owing to weak localization and Coulomb interaction effects. The black straight lines highlight this behaviour. Transition temperatures equal to 1.3, 1.0 and 0.45 K for TiN1, TiN2 and TiN3, respectively, are obtained by fitting the conductance curves with all the quantum corrections to the conductivity. The fitting procedure is described in the Methods. The fits are shown as solid curves. Full size image The enhanced electron–electron interactions manifest themselves not only in the observed suppression of T c in TiN films but, further, also in the insulating trend in the resistance. This is illustrated in Figure 1b in which, in order to stress that in TiN films the distinct insulating behaviour is clearly seen even at room temperature, we have plotted the inverse resistance 1/ R as function of temperature. Pseudogap in the DOS The most direct access to the gap in the electronic excitation spectrum is offered by scanning tunnelling microscope (STM) probe measuring tunnelling conductance G . The DOS, ν ( η ), is found as a function of the single-electron excitation energy (relative to the Fermi level), η = E − E F , and of the temperature T by recording the differential conductance G ( V )=d I /d V of the tunnelling junction between the STM tip and the sample versus its voltage bias V . The tunnelling conductance relates to ν ( η ) by where f T is the Fermi distribution function at temperature T (ref. 5 ). We probed the tunnelling conductance of superconducting films TiN1, TiN2 and TiN3, with a STM cooled down in a dilution refrigerator. 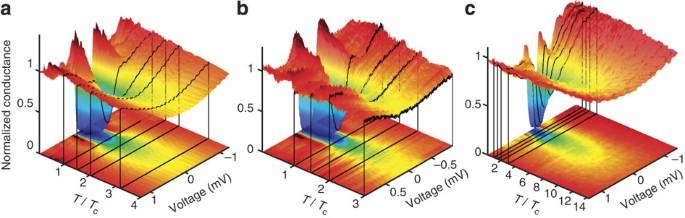Figure 2: Pseudogap in the density of states. Three-dimensional plots of the tunnelling conductanceG(V,T/Tc) normalized by the conductance measured at high voltage and low temperature as a function of bias voltage and normalized temperatureT/Tcfor superconducting films TiN1 (a), TiN2 (b) and TiN3 (c). Black lines mark the spectra measured atT/Tc=1, 1.5, 2 and 3, illustrating that the pseudogap state grows more pronounced and extends over a wider temperature range as the disorder increases. The suppression of the density of states of the TiN3 sample remains visible up toT=14Tc. Importantly, the transport measurements of the resistance of films TiN1, TiN2 and TiN3, shown in Figure 1 , and STM, displayed in Figure 2 , were carried out during the same run. At the lowest temperatures, all three samples display a gap centred at the Fermi level, corresponding to zero bias, V =0, and two peaks at the edges of the gap, in accordance with the Bardeen–Cooper–Schrieffer theory of conventional s -wave superconductivity [1] , as observed in our previous work [22] . On increasing temperature, the gap gets shallower and coherence peaks are depressed. However, up to the maximal temperatures achievable in our experiments, the suppression in the DOS remains substantial. Moreover, while approaching the critical disorder strength at which the disorder-driven SIT occurs, both the depth of the pseudogap and the temperature range in which it exists, show the trend to increase. Remarkably, the pronounced pseudogap persists up to 6.3 K, the highest temperature achieved in the experiment, which is ~14 T c for the TiN3 sample. At variance, in a 100-nm-thick TiN film, which is well within the three-dimensional domain with respect to superconducting properties, a flat metallic DOS is restored exactly at T c (see ref. 23 ). Figure 2: Pseudogap in the density of states. Three-dimensional plots of the tunnelling conductance G ( V , T / T c ) normalized by the conductance measured at high voltage and low temperature as a function of bias voltage and normalized temperature T/T c for superconducting films TiN1 ( a ), TiN2 ( b ) and TiN3 ( c ). Black lines mark the spectra measured at T/T c =1, 1.5, 2 and 3, illustrating that the pseudogap state grows more pronounced and extends over a wider temperature range as the disorder increases. The suppression of the density of states of the TiN3 sample remains visible up to T =14 T c . Full size image Superconductivity-related origin of the pseudogap To uncover the nature of the observed pseudogap, we juxtapose the direct STM observations of the DOS with the results of our parallel measurements of the transport conductance. Figure 1b shows the T -dependence of the dimensionless conductance g =( h / e 2 R ) in a semi-logarithmic scale. In all samples, it decreases logarithmically on cooling from room temperature down to ~10 K, as expected for two-dimensional disordered metals described by the standard theory of quantum corrections to conductivity. This behaviour reflects that predominating contributions stem from quantum interference effects, namely, weak localization, and electron–electron interaction [24] , [25] , [26] . In the superconducting samples, the noticeable deviation from the logarithmic dependence takes place on approaching T c (see Methods). The main contribution to the conductance upturn comes from SFs (ref. 27 ). Their role is twofold: to organize Cooper pairs, the part of the electronic states should be borrowed from the normal metal, leading to a suppression of the metallic DOS. It results in an insulating trend in the temperature dependence of the resistance, which, thus, grows on decreasing temperature. At the same time, fluctuation-induced Cooper pairs short circuit electronic conductivity, and, as the SFs become developed enough, this shunting effect disguises the suppressing of the DOS. A corresponding temperature evolution of the SF-induced suppression of DOS and the resulting change in the tunnelling conductance has been discussed by Varlamov and Dorin [28] within the framework of the perturbation theory of SFs [27] and is described by the 'double-log' temperature dependence: where ɛ =ln( T/T c ) is the reduced temperature. To relate the observed pseudogap to SFs, we inspect the measured temperature evolution of the differential tunnelling conductance at zero bias. 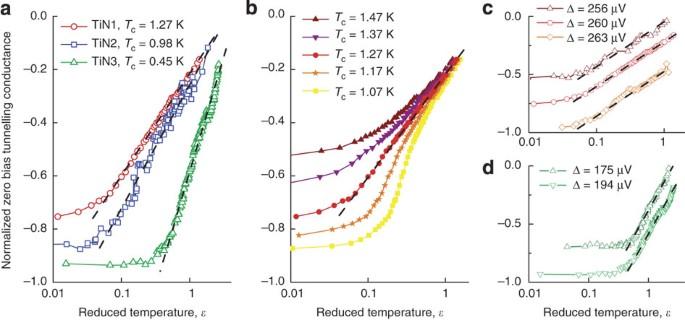Figure 3: Temperature dependence of the zero-bias tunnelling conductance. The thermal evolution of the normalized differential conductanceδG/G=(G(V=0,ɛ)−G0)/G0, whereG0is the differential conductance at high voltage and high temperature, is represented as a function of the reduced temperatureɛ=ln(T/Tc) in semi-logarithmic plots. (a) The dashed straight lines accentuate the double-logarithmic temperature dependence (that is, as function of ln[ln(T/Tc)]) of the pseudogap at the Fermi level for each of the three samples. (b) Illustration of the no-fitting-parameter character of our plots, for the case of TiN1. Even the slight modification ofTcwould have eliminated the linear dependence ofδG/Gon ln[ln(T/Tc)]. (c,d) Independence of the double-logarithmic temperature behaviour on the position at which the local superconducting gap Δ is measured atT≪Tc. The spatial fluctuations of Δ observed in ref.22do not affect the double-logarithmic temperature behaviour as shown for TiN1 (c) and TiN3 (d). The curves are shifted for clarity. As shown in Figure 3a , the raw data follow equation (2) with the high accuracy over a wide range of reduced temperature, ɛ, and the slopes of δG ( V =0, ɛ ) versus ln ɛ dependences increase with disorder, that is, with R . It is noteworthy that the plots do not contain any adjusting parameter: the value of T c is independently derived from the transport measurements data (see Methods and Supplementary Fig. S1 ). At the same time, δG ( V =0, ɛ ) versus ln ɛ dependence offers an independent method for determining T c . Indeed, the slightest change in T c eliminates the linear dependence of δG ( V =0, ɛ ) on ln ɛ , as seen in Figure 3b . This dependence holds over a wide temperature range only when correct, within the 50 mK accuracy, critical temperature, T c , is chosen, evidencing a remarkable consistency between the local spectroscopic measurements and the macroscopic transport data, irrespective of the spatial fluctuation of the gap amplitude observed in ref. 22 (see Fig. 3c,d ). However, it must be noted that the maximum energy differences in gap values observed at very low temperature are only of a few tens of microelectron volts. At higher temperature, in the pseudogap state, these energy differences are likely to be washed out and, in any case, are beyond the energetic resolution of tunnelling spectroscopy, owing to the large thermal smearing. Figure 3: Temperature dependence of the zero-bias tunnelling conductance. The thermal evolution of the normalized differential conductance δG/G =( G ( V =0, ɛ )− G 0 )/ G 0 , where G 0 is the differential conductance at high voltage and high temperature, is represented as a function of the reduced temperature ɛ =ln( T/T c ) in semi-logarithmic plots. ( a ) The dashed straight lines accentuate the double-logarithmic temperature dependence (that is, as function of ln[ln( T/T c )]) of the pseudogap at the Fermi level for each of the three samples. ( b ) Illustration of the no-fitting-parameter character of our plots, for the case of TiN1. Even the slight modification of T c would have eliminated the linear dependence of δG / G on ln[ln( T/T c )]. ( c , d ) Independence of the double-logarithmic temperature behaviour on the position at which the local superconducting gap Δ is measured at T ≪ T c . The spatial fluctuations of Δ observed in ref. 22 do not affect the double-logarithmic temperature behaviour as shown for TiN1 ( c ) and TiN3 ( d ). The curves are shifted for clarity. Full size image Equation (2) holds over the whole domain of Gaussian fluctuations, Gi ≪ ɛ ≪ 1, as long as the condition δG/G ≪ 1 is satisfied. At the same time, Figure 3 shows that the ln ɛ law describes the experimental data fairly well, even beyond the perturbative regime extending to the region in which the SF corrections are large, and also persists to well above T c , where ɛ ≥1. The limit, Gi ≪ 1, determines the temperature below which one enters the critical region where the fluctuations are correlated and cannot be any longer considered as Gaussian. In Figure 3 , this corresponds to plateaus in which the DOS is nearly temperature independent. As expected from the SF theory [27] , both, the temperature range of this critical regime as well as the slope of the ln[ln( T/T c )] dependence, increase from the less resistive sample TiN1 to the more resistive one TiN3, reflecting the increase of Gi with disorder. These results indicate that the origin of the observed pseudogap in TiN film is the suppression of DOS by two-dimensional SFs. To conclusively rule out other possibilities, we inspected the role of Coulomb interactions, which, in principle, contribute to the suppression of the DOS (refs [24] , [25] , [26] 24–26), resulting in the so-called Aronov–Altshuler–Lee zero-bias anomaly. The Coulomb effects lead to the logarithmic behaviour of the transport conductance at temperatures not too close to T c , as shown in Figure 1b . However, re-plotting the tunnelling conductance above T c , shown in Figure 3a , as function of ln T , does not reveal a linear dependence of G on ln T . Thus, the zero-bias anomaly does not influence the DOS near T c , which is not unexpected: in the close vicinity of superconducting transition, the SF-induced double-logarithmic divergence of the tunnelling conductance is by far stronger. Incidentally, our findings show that SFs not only dominate the DOS behaviour at E F but also govern the transport properties at very low voltages. A key question in pseudogap studies is whether the pseudogap phenomenon is due to an exotic electronic structure of the cuprates and the related non-conventional mechanisms of superconductivity or is a generic property of a wide class of superconducting materials. As a matter of fact, Nernst effect [29] and magnetization measurements [30] in these systems have unveiled superconducting phase fluctuations, whose importance is still debated [31] . Our findings reveal that the SF-dominated temperature region in the ultrathin TiN films extends to temperatures well above T c , with a striking resemblance to the behaviour of the copper oxides. The SF-induced pseudogap persists up to 6.3 K, the highest temperature achieved in the experiment, which is ~14 T c for the sample with maximally suppressed T c . This demonstrates another strong parallel between high-temperature superconductors and thin films of conventional superconductors, namely, the extension of the temperature range in which the pseudogap state has been observed on approaching the SIT. The conclusion to be drawn is that the quantitative analysis of our data establishes unambiguously the existence and origin of the pseudogap state in ultrathin films of conventional superconductors. The pseudogap there results from quasi-two-dimensional SFs suppressing the DOS, and is further enhanced by the proximity to the SIT. Given that cuprates are comprised of conducting Cu-O planes, thus bringing in the two-dimensional effects, our findings offer new insight into a fascinating pseudogap state in high-temperature superconductors, suggesting that quasi-two-dimensional SFs may have a primary role in its formation. This calls for the similar quantitative analysis of the fluctuation-related phenomena in cuprates, in order to evaluate the actual importance of two-dimensional fluctuation effects in the pseudogap of these materials. Such an analysis may therefore become a decisive component in disentangling SFs effects from other possible contributions in the long-standing mystery of the pseudogap state. Sample preparation Our samples are ultrathin films of TiN synthesized by atomic-layer chemical deposition onto a Si/SiO 2 substrate. TiN1 is a 3.6-nm-thick film deposited at 400 °C, whereas TiN2 and TiN3 are 5.0-nm-thick films deposited at 350 °C. TiN3 was then slightly plasma etched to reduce its thickness. Electron transmission and diffraction pattern revealed the films to be made of densely packed crystallites with a typical size of 5.0 nm. Samples were patterned into Hall bridges using conventional ultraviolet lithography and plasma etching. Well below T c , they display a disorder-induced inhomogeneous superconducting state revealed by scanning tunnelling spectroscopy performed at 50 mK [22] . Measurements The STM Pt/Ir tip was aligned above one of the free 500×500 μm 2 contact pads of the Hall bridge. To probe the local DOS, the differential conductance of the tunnel junction, G ( V )=d I /d V , was measured by a lock-in amplifier technique, with an alternative voltage of 10 μV added to the ramped bias voltage. The tunnelling current was 0.5–1.0 nA for milliVolts bias voltage, yielding a tunnelling resistance of ~1–2 MΩ, which is much higher than the sheet resistance of our samples. Hence, no voltage drop across the resistive film in series with the STM junction occurs during spectroscopy. Four probe measurements of the film resistance were carried out by acquiring both voltage and current with a low-frequency lock-in amplifier technique in a four terminal configuration. Transport measurements and tunnelling spectroscopy were systematically carried out during the same run in a home-built STM cooled down to 50 mK in a dilution refrigerator. Temperature of the sample holder, which was weakly coupled to the dilution refrigerator, was accurately controlled by a RuO 2 thermometer and a resistive heater. It is worth noticing that no measurable thermal drift of the tip position occurs in our STM between the base temperature of 50 mK and the highest measured temperature of ~6.3 K. Quantum corrections to the conductivity and determination of T c The fundamentals of the theory of quantum corrections to the conductivity of disordered metals can be summarized as follows [24] , [27] , [32] , [33] : first, the diffusive motion of a single electron is accompanied by the quantum interference of the electron waves (the effect is referred to as the weak localization (WL)); second, in disordered systems, the electron–electron interactions (EEI) increase. These effects result in so-called quantum corrections to the classical Drude conductivity G 0 , yielding the following form of the total conductivity: Quantum corrections stemming from the electron–electron interaction comprise, in their turn, two parts. A correction of the first type, known as the interaction in a diffusion channel (ID), involves the interaction between particles with close momenta. A second type correction is the quantum correction originating from the electron–electron interaction in the Cooper channel, in which the total momentum of interacting electrons is small. This correction is essential in the systems crossing over to the superconducting state and is referred to as the fluctuational superconductivity. The corrections to the conductivity caused by the fluctuation-induced formation of Cooper pairs or, which is the same, by the interaction in the Cooper channel branch into three distinct types. The first one is the famous Aslamazov–Larkin term (AL) describing the direct contribution of SFs to conductivity, that is, the flickering short circuiting of conductivity by the fluctuating Cooper pairs. The second type of conductivity corrections appear because, in order to form the fluctuation Cooper pairs above T c , some of the normal electron states have to be borrowed. This results in some depression of the normal excitations' DOS or, equivalently, in an effective decrease in the number of normal conducting electrons. According to the Drude formula, this leads to the decrease in the normal electron conductivity. This contribution is known as the DOS suppression term. The third type correction is the Maki–Thompson correction (MT) coming from the coherent scattering of impurities of the electrons forming a Cooper pair. In terms of these corrections, the total conductivity acquires the form: In quasi-two-dimensional disordered superconducting systems, where the thickness d of a superconducting film is larger than both, the Fermi wavelength, λ F , and the mean free path, l , but is less than the lengths responsible for the electron–electron interaction in both the Cooper channel ( ξ —the superconducting coherence length) and the diffusion channel is the thermal coherence length), that is, λ F , l < d < ξ , L T , these corrections cast into the following: where G 00 = e 2 /(2 π 2 ħ). where B =ln{2 π /[ e 2 R ln( π /( e 2 R ))]} ( R is the resistance per square) and β ( T/T c ) is the electron–electron interaction strength function introduced and tabulated by Larkin [32] : The temperature dependencies corresponding to the corrections calculated from equations (5) to (8) together with the curve describing the sum of all the corrections are shown in Supplementary Figure S1 by solid lines. The experimental data are shown as yellow-filled circles. The alignment of the theoretical curves and the experimental data was carried out at the reference point 10 K according to formula: The fitting parameters here are the coefficient A from equation (5) and T c . One immediately notes that down to the temperature T = T SF , where T SF ≈7.2 K, T SF ≈5.7 K and T SF ≈2.9 K for samples TiN1, TiN2 and TiN3, respectively, the contributions to the resistance from superconducting fluctuating corrections, Δ G AL , Δ G DOS and Δ G MT , all compensate each other (in the determination of these temperatures, the criterion that the divergence of the curve corresponding to the sum of all corrections and the curve corresponding to the WL+ID contributions only was 1%). Therefore, at temperatures above T SF , the resistance curves follow the temperature dependencies defined by Δ G WL ( T )+Δ G ID ( T ). This is the reason why SFs at high temperatures are hardly detectable by conductance measurements, but can be observed by tunnelling spectroscopy, which specifically probes the DOS correction. At lower temperatures, Δ G MT ( T ) dominates the temperature behaviour of the resistance and the corresponding curve bends down. When fitting the data, for R , entering the parameter B , its value at 10 K was taken. Importantly, the fitting parameters A and T c are determined independently: A is found from the fit in the 'high'-temperature interval from predominantly WL+ID correction curve, whereas T c is determined from the fit at lower temperatures in the Maki–Thompson-dominated domain. This ensures the high precision determination of T c presented in Supplementary Table S1 . How to cite this article: Sacépé, B. et al . Pseudogap in a thin film of a conventional superconductor. Nat. Commun. 1:140 doi: 10.1038/ncomms1140 (2010).